Induction and control of supramolecular chirality by light in self-assembled helical nanostructures Evolution of supramolecular chirality from self-assembly of achiral compounds and control over its handedness is closely related to the evolution of life and development of supramolecular materials with desired handedness. Here we report a system where the entire process of induction, control and locking of supramolecular chirality can be manipulated by light. Combination of triphenylamine and diacetylene moieties in the molecular structure allows photoinduced self-assembly of the molecule into helical aggregates in a chlorinated solvent by visible light and covalent fixation of the aggregate via photopolymerization by ultraviolet light, respectively. By using visible circularly polarized light, the supramolecular chirality of the resulting aggregates is selectively and reversibly controlled by its rotational direction, and the desired supramolecular chirality can be arrested by irradiation with ultraviolet circularly polarized light. This methodology opens a route to ward the formation of supramolecular chiral conducting nanostructures from the self-assembly of achiral molecules. Circularly polarized light (CPL) is considered to be a true chiral entity and has been attributed as the origin of the homochirality of biological molecules [1] , [2] , as chiral information encoded in CPL can be transferred to molecules. Irradiation with CPL of a racemic mixture of chiral molecules can selectively enrich one enantiomer up to a small extent, called ‘symmetry breaking’ [3] , [4] . It has been speculated that this slight chiral bias might have been amplified via autocatalytic reactions or crystallization processes during the evolutionary process [5] , resulting in homochirality. Amplification of the chiral information and macroscopic expression of chirality has been observed with liquid crystals, where the excess enantiomer generated by CPL acts as a chiral dopant and induces a chiral liquid crystalline phase [6] , [7] , [8] . Chiral information in CPL could be also transferred to helical polymers and expressed at a secondary structure level, as the handedness of the helix was controlled by the direction of CPL [9] , [10] , [11] . Supramolecular chirality has been generally induced by the self-assembly of homochiral molecules or a mixture of chiral and achiral molecules, where the molecular chirality is transferred (and amplified as well in case of the mixture) to the handedness of the self-assembled helical structure [12] , [13] , [14] , [15] . Only a few papers have described generation of supramolecular chirality by irradiation of azobenzene-containing achiral molecules with CPL, presumably through alignment of the azobenzene chromophores following the direction of CPL [16] , [17] , [18] . In contrast to the preceding research, here we apply CPL to a light-induced self-assembly process so that the CPL irradiation triggers the self-assembly and simultaneously transfers the chiral information to the self-assembled structure. As a key molecular motif for the light-induced self-assembly process, we use a triphenylamine (TPA) moiety that contains three phenyl rings connected to a central nitrogen atom similar to the blades of a propeller. TPA-containing molecules have been shown to self-assemble on light exposure in chlorinated solvents by the formation of triphenylammonium radicals that adopt more planar configurations than the neutral forms and facilitate stacking [19] , [20] , [21] , [22] , [23] . Simply by employing CPL as a light source in the self-assembly process of a TPA-containing molecule, we show that self-assembled aggregates with supramolecular chirality can be generated, driven by the helical stacking of the TPA moieties. Our data suggest that the chiral bias generated by irradiation of the TPA moiety with CPL is amplified by the self-assembly process, which promotes enrichment of one enantiomer by the enantioselective helical stacking and forms aggregates with specific handedness. The handedness of the aggregates is exclusively dictated by the rotational direction of the CPL and can even be switched in a totally reversible manner. Furthermore, by incorporating a diacetylene (DA) moiety that undergoes topochemical photopolymerization by ultraviolet (254 nm) [24] , [25] , we demonstrate that the desired handedness can be permanently locked by circularly polarized ultraviolet light (CPUL) irradiation, which knits the self-assembled structure with covalent bonds [26] , [27] , [28] . We believe this to be the first example of light-induced self-assembling systems where the entire process of induction, control and locking of supramolecular chirality can be solely manipulated by CPL. Synthesis and photoinduced self-assembly Achiral compound 1 was synthesized by amide coupling reaction between an amine-functionalized TPA molecule ( 2 ) and a carboxylic acid-functionalized DA molecule ( 3 ) as shown in Fig. 1 . 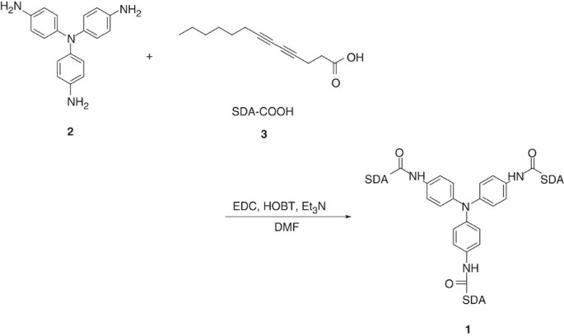Figure 1: Synthesis of the compound1. The achiral compound1consisting of the TPA moiety in the centre and the diacetylene units at the periphery was synthesized by amide coupling reaction between a TPA-containing molecule2and a diacetylene-containing molecule3. Figure 1: Synthesis of the compound 1 . The achiral compound 1 consisting of the TPA moiety in the centre and the diacetylene units at the periphery was synthesized by amide coupling reaction between a TPA-containing molecule 2 and a diacetylene-containing molecule 3 . Full size image Although the 1 H nuclear magnetic resonance (NMR) spectrum of 1 in deuterated dimethyl sulfoxide (DMSO- d 6 ) showed clearly resolved aromatic and amide protons, irradiating with light from a fluorescent lamp for a few minutes on deuterated 1,2-dichloroethane (DCE- d 4 ) solution of 1 turned the colour of the solution from orange to green and its 1 H NMR spectrum revealed no signal in the 6–11 p.p.m. range where the aromatic and amide protons should appear ( Supplementary Fig. 1 ). This observation, consistent with the literature [20] , [21] , [22] , [29] , indicates that a small number of triphenylammonium radicals were generated by light exposure and triggered stacking of the TPA moieties with the aid of amide hydrogen bonding. Chlorinated solvents seem to play an important role in the radical generation process, as solvent radicals are easily formed by light exposure, and reversibly transfer electrons to the TPA moiety. Formation of the triphenylammonium radicals is believed to facilitate stacking of the radicals, as π – π interaction between the radicals becomes effective as they adopt a more planar configuration and electric interaction of the radical cation–anion pairs further stabilizes the stack. Simulation of a TPA-containing molecule similar to 1 suggests that the energy gain for the neutral precursor by joining the stack is greater than the energy penalty for the required configuration change to a more planar form; thus, eventually self-assembled aggregates containing a small number of triphenylammonium radicals would be generated. The photoinduced self-assembly of 1 was observed in various chlorinated solvents and the morphology was visualized by field-emission scanning electron microscopy (FE-SEM) after evaporation of the solvent. 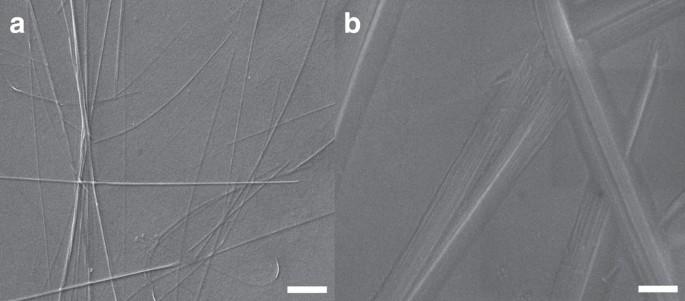Figure 2: Fibrillar aggregates formed by light irradiation. FE-SEM images of the aggregates of1formed in DCE solution (2 mg ml−1concentration) by visible light irradiation. The sample was coated with Au before imaging. (a) Low magnification. Scale bar, 10 μm. (b) High magnification. Scale bar, 500 nm. Figure 2 shows the self-assembled structure of 1 formed in DCE, revealing fibrillar aggregates with several tens of micrometres in length and an average diameter of 980 (±180) nm. A close look indicated that the fibril was composed of bundles of nanofibres with diameters of ca . 23 (±4.9) nm, which is consistent with the transmission electron microscopy images of the aggregates ( Supplementary Fig. 2a ). For comparison, an FE-SEM image of a sample prepared without light exposure showed no distinct morphology, suggesting stacking of the TPA moieties triggered by light exposure is important in the formation of the one-dimensional self-assembled structure ( Supplementary Fig. 2b ). Figure 2: Fibrillar aggregates formed by light irradiation. FE-SEM images of the aggregates of 1 formed in DCE solution (2 mg ml −1 concentration) by visible light irradiation. The sample was coated with Au before imaging. ( a ) Low magnification. Scale bar, 10 μm. ( b ) High magnification. Scale bar, 500 nm. Full size image An X-ray diffraction (XRD) pattern of the solid obtained by the photoinduced self-assembly exhibited a single broad peak at 2 θ =21° corresponding to spacing ( d ) of 0.42 nm, which is attributed to the intermolecular distance between stacked TPA moieties ( Supplementary Fig. 3a ). Appearance of the diffraction peaks in the small-angle regime also indicates periodicity of the aggregates at a nanometre-length scale ( Supplementary Fig. 3b ). We consider the peak at 2 θ =3.0° in particular corresponds to d =2.94 nm, originating from the distance between the stacks, assuming the intercalation of alkyl groups. Second- and third-order diffractions at 2 θ =6.0° and 9.2° were also observed. Assuming a hexagonal geometry, the peak at 2 θ =5.5° and 8.1° may be assigned as √3 and √7 diffractions. We also note that a similar TPA-containing molecule with long alkyl chains without DA moieties has been shown to form self-assembled nanofibres in solution, presumably by alkyl chain packing and amide hydrogen bonding, resulting in physical gelation of the solvent [30] . The existence of amide hydrogen bonding was also observed in our system by attenuated total reflection infrared spectroscopy of 1 after light irradiation and evaporation of solvent ( Supplementary Fig. 4 ) [22] , [30] , [31] . The self-assembled structure of 1 was estimated by computation based on density functional theory (DFT). To properly predict the most thermodynamically stable structure, ω B97X-D functional and 6–31G* basis set were used to approximate the electron density and molecular interactions of the self-assembled structure composed of large numbers of atoms [32] . 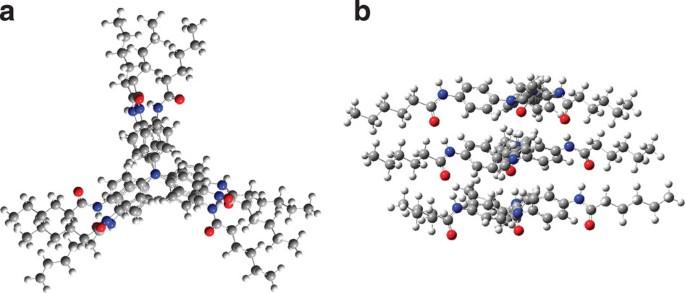Figure 3: Self-assembled structure of1estimated by calculation. The self-assembled structure of1(trimer) was calculated by DFT method. The molecular structure was simplified by substituting the side chains withn-pentyl groups. Images were taken from the top (a) and the side (b) of the stacks. Figure 3 depicts an optimized trimer obtained with a simplified molecular structure, suggesting that 1 self-assembles into helical stacks via hydrogen bonding of the amides (see Methods and Supplementary Fig. 5 for calculation details). The structure resembles the C3 symmetric helical supramolecular structures based on 1,3,5-benzenetricarboxylic acid and others thoroughly studied by Meijer and colleagues [33] , [34] , [35] . Figure 3: Self-assembled structure of 1 estimated by calculation. The self-assembled structure of 1 (trimer) was calculated by DFT method. The molecular structure was simplified by substituting the side chains with n -pentyl groups. Images were taken from the top ( a ) and the side ( b ) of the stacks. Full size image Induction and control of supramolecular chirality by CPL When a normal light was used for the radical generation process, the solution after irradiation showed no circular dichroism (CD) activity, suggesting that it contained a racemic mixture of both left- and right-handed helical aggregates of 1 . However, irradiation of the DCE solution of 1 with l -CPL produced intense CD activity with two positive maxima at 222 and 319 nm, and two negative maxima at 240 and 360 nm ( Fig. 4a ). The intensity increased over irradiation time and became level after 10 min ( Fig. 4b ). 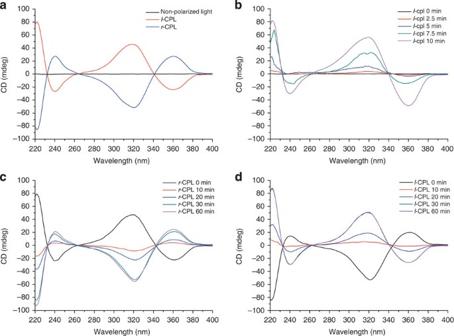Figure 4: Induction and control of supramolecular chirality by CPL. CD spectra of1in DCE solution after irradiation with CPL. (a) Spectra after irradiation with non-polarized light (black),l-CPL (red) andr-CPL (blue) for 10 min. (b) Time-dependent evolution of CD activity on irradiation withl-CPL. (c) Inversion of CD activity by irradiation withr-CPL of the solution that had been pre-exposed tol-CPL. (d) Inversion of CD activity by irradiation withl-CPL of the solution that had been pre-exposed tor-CPL. Figure 4: Induction and control of supramolecular chirality by CPL. CD spectra of 1 in DCE solution after irradiation with CPL. ( a ) Spectra after irradiation with non-polarized light (black), l -CPL (red) and r -CPL (blue) for 10 min. ( b ) Time-dependent evolution of CD activity on irradiation with l -CPL. ( c ) Inversion of CD activity by irradiation with r -CPL of the solution that had been pre-exposed to l -CPL. ( d ) Inversion of CD activity by irradiation with l -CPL of the solution that had been pre-exposed to r -CPL. Full size image The use of r -CPL produced the exact identical result, except with the opposite sign of CD activity, suggesting that helical aggregates with a desired handedness can be selectively generated by choice of the rotational direction of CPL [36] , [37] . More interestingly, the supramolecular chirality generated by l - or r -CPL could be reversibly switched by irradiation with the CPL of the opposite rotational direction. For instance, time-dependent CD activity change was monitored during irradiation of r -CPL on the DCE solution of 1 , which had been pre-irradiated by l -CPL ( Fig. 4c ). The initial CD activity generated by l -CPL was rapidly suppressed after 10 min of exposure, whereas the CD activity of the opposite sign evolved over time and reached the maximal value after 60 min. The maximal intensity achieved after 60 min was identical to the value that was obtained by irradiation of r -CPL on the unexposed solution to light, indicating full inversion of supramolecular chirality. As expected, chirality inversion by l -CPL produced the exactly identical result, except with the opposite direction of CD activity change ( Fig. 4d ). The inversion process could be reversibly repeated without any sign of loss of optical activity ( Supplementary Fig. 7 ), but irradiation with non-polarized light decreased CD activity over time ( Supplementary Fig. 8 ). Although there has been no literature reporting the generation of supramolecular chirality using the TPA moiety, we suggest that irradiation with CPL induces radical formation at the nitrogen atom of the TPA moiety and also generates preferential chiral arrangements of the phenyl rings. As illustrated by the DFT calculation results, the phenyl rings in the TPA radical would be twisted with respect to the C3 symmetric plane resembling the blades of a propeller. We posit that the interaction of π electrons in the phenyl rings with the angular momentum of CPL would determine the preferential twisting direction by photoresolution effect [38] to produce the TPA moiety with a certain enantiomeric form. ‘Enantioselective’ stacking of the TPA moieties possessing phenyl rings with the identical twisting direction should result in helical aggregates with one handedness. Simulation of CD spectra of the estimated self-assembled structure by DFT calculation suggests that indeed such a stacking structure can generate CD activity, which was qualitatively in agreement consistent with the experimental data, and l -CPL and r -CPL (as defined from the point of view of the receiver) produce left-handed and right-handed helicity, respectively ( Supplementary Fig. 6 ). Chiral asymmetry would be more amplified, because only the TPA moieties with the same arrangements (that is, same enantiomer) would participate in the self-assembly process and be stabilized by the enthalpic gain. The fact that the evolution of CD activity on CPL irradiation was faster on the unexposed solution than the solution pre-irradiated by CPL suggests the process of supramolecular chirality inversion would include reversible dissociation of terminal molecules of a helical aggregate, chirality inversion at a molecular level and nucleation/growth of the helical aggregate with opposite handedness [39] , [40] , [41] . Locking of supramolecular chirality by photopolymerization As noted above, the generated supramolecular chirality disappears under exposure to non-CPL such as ambient light from a common fluorescent lamp on the ceiling ( Supplementary Fig. 8 ). To permanently lock the supramolecular chirality, we exploited the photopolymerization of DA moieties, by applying ultraviolet irradiation (254 nm, non-polarized) to the DCE solution of 1 , which had been pre-irradiated with visible light and consisted of self-assembled aggregates. The photopolymerizability of the self-assembled structure was verified by Fourier transform (FT) Raman spectroscopy with an excitation wavelength of 633 nm. The sample obtained by spin coating of the ultraviolet-irradiated solution on glass showed clearly discernable peaks at 1,492 and 2,113 cm −1 corresponding to ν (C=C) and ν (C≡C), respectively, of the conjugated DA polymer, indicating successful polymerization of DA ( Fig. 5a ) [42] , [43] . The broad background peak was attributed to the inherent fluorescence from the TPA moiety [44] , [45] . 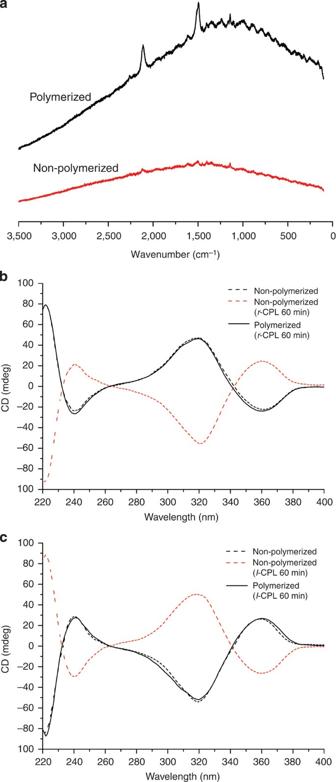Figure 5: Locking of supramolecular chirality by photopolymerization. (a) Fourier-transform Raman (FT-Raman) spectra of spin-coated films of DCE solution of1on glass. Film prepared after photopolymerization in solution (black solid line). Film prepared without polymerization (red solid line). (b,c) Persistence of CD activity of DCE solution of1after photopolymerization by CPUL against inversion by irradiation with CPL of the opposite rotational direction. The polymerized aggregate obtained by sequential irradiation with CPL and CPUL of the identical rotational direction possesses permanent handedness. Notice that the CD spectrum of the polymerized sample (black solid line) does not change its CD activity on irradiation with CPL of the opposite rotation direction for 60 min; the spectrum almost completely overlaps the original CD spectrum of the sample before photopolymerization (black dashed line). For comparison, inversion of CD activity of the non-polymerized sample on irradiation with CPL of the opposite direction was also shown (red dashed line, same data fromFig. 4). (b) Spectra of1polymerized withl-CPUL and then exposed tor-CPL (black solid line). Spectra of non-polymerized1after irradiation withl-CPL (black dashed line) and then exposed tor-CPL (red dashed line) are also shown. (c) Spectra of1obtained with CPL and CPUL of the opposite rotational direction. Figure 5: Locking of supramolecular chirality by photopolymerization. ( a ) Fourier-transform Raman (FT-Raman) spectra of spin-coated films of DCE solution of 1 on glass. Film prepared after photopolymerization in solution (black solid line). Film prepared without polymerization (red solid line). ( b , c ) Persistence of CD activity of DCE solution of 1 after photopolymerization by CPUL against inversion by irradiation with CPL of the opposite rotational direction. The polymerized aggregate obtained by sequential irradiation with CPL and CPUL of the identical rotational direction possesses permanent handedness. Notice that the CD spectrum of the polymerized sample (black solid line) does not change its CD activity on irradiation with CPL of the opposite rotation direction for 60 min; the spectrum almost completely overlaps the original CD spectrum of the sample before photopolymerization (black dashed line). For comparison, inversion of CD activity of the non-polymerized sample on irradiation with CPL of the opposite direction was also shown (red dashed line, same data from Fig. 4 ). ( b ) Spectra of 1 polymerized with l -CPUL and then exposed to r -CPL (black solid line). Spectra of non-polymerized 1 after irradiation with l -CPL (black dashed line) and then exposed to r -CPL (red dashed line) are also shown. ( c ) Spectra of 1 obtained with CPL and CPUL of the opposite rotational direction. Full size image As a comparison, a sample not exposed to ultraviolet radiation exhibited almost no intensity at the characteristic vibration frequencies for the conjugated DA polymer. The result suggests that only preorganized DA moieties in the self-assembled structure can undergo topochemical polymerization, which requires an optimal and long-range arrangement of adjacent DA moieties. Stability of the polymerized assembly was also evaluated by dynamic light scattering analysis. Although the polymerized sample maintained its scattering intensity in DCE as well as in DMSO, the non-polymerized sample showed no scattering intensity in DMSO, indicating dissolution of the assembly into individual molecules ( Supplementary Fig. 9 ). SEM imaging did not reveal particular changes in the morphology of the aggregates after polymerization ( Supplementary Fig. 10 ). XRD patterns of the polymerized sample were also similar to that of non-polymerized one, but showed more refined peaks in the small-angle regime, suggesting increased periodicity between stacks by polymerization of DA moieties ( Supplementary Fig. 3c,d ). We envision that lateral ordering of the alkyl chains would be self-corrected by topochemical polymerization to form more regular stacks. In addition, formation of a new C–C bond per alkyl chain by the polymerization would restrict mobility of the alkyl chains and stiffen the covalently joined stacks, resulting in the more well-ordered packing of the stacks. The diffraction peaks in the wide-angle regime did not show a noticeable difference, suggesting aromatic packing was not affected by polymerization. However, the use of non-polarized ultraviolet induced racemization of the self-assembled structure resulting in the polymerized assembly with no CD activity. To maintain the desired handedness during the photopolymerization process, we employed CPUL. Irradiation of the DCE solution of 1 with CPL and subsequent irradiation with CPUL of the same rotational direction produced polymerized aggregates with controlled handedness, corresponding to the rotational direction of the polarized light. The CD activity was completely retained, suggesting the helical arrangement was not affected by polymerization. Moreover, the polymerized aggregates showed remarkable stability against inversion of supramolecular chirality on irradiation with CPL of the opposite rotational direction. In contrast to non-polymerized aggregates that changed their handedness completely after 60 min of CPL irradiation with the opposite rotational direction, the polymerized aggregates showed no sign of CD activity change on irradiation ( Fig. 5b,c ). The result clearly indicates photopolymerization of the DA moieties by CPUL successfully locked the supramolecular chirality. We also tested whether the polymerized aggregate with certain handedness could nucleate further stacking of 1 , following its handedness, under non-CPL irradiation. However, we observed that the CD activity as well as the particle size did not noticeably increase after the non-CPL irradiation, indicating that new aggregates were formed with a 50:50 population of both handedness ( Supplementary Fig. 11a ). It seems that the aggregate end may adopt a slightly different configuration and the enthalpic gain obtained by interaction of 1 and the aggregate end may not be greater than between 1 . The whole process of induction, control and locking of supramolecular chirality by CPL and CPUL is summarized in Fig. 6 . Irradiation with r - or l -CPL induces self-assembly of 1 in chlorinated solution and control over handedness of the forming helical aggregates. The resulting handedness is totally switchable by irradiating with CPL of the opposite rotational direction. Subsequent irradiation with CPUL of the identical rotational direction polymerizes adjacent DA moieties, to convert the self-assembled aggregate into a covalently joined nano-object, and permanently locks the handedness. To our knowledge, this is the first example of controlling and fixing supramolecular chirality from an achiral compound by light. 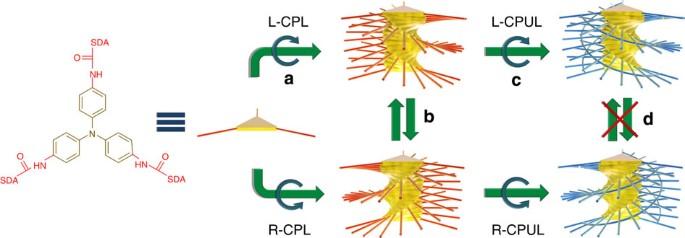Figure 6: Manipulation of supramolecular chirality entirely by light. The whole process of induction, control and locking of supramolecular chirality by CPL and CPUL from an achiral compound1containing TPA (yellow) and DA (red: non-polymerized, blue: polymerized) moieties is schematically depicted. Irradiation with CPL induces self-assembly of1with control over handedness (a) and the handedness can be reversibly switched by irradiating with the counter CPL (b). Photopolymerization of the DA moieties by CPUL irradiation knits the self-assembled structure to produce a covalently joined nano-object (c) and the supramolecular chirality is permanently locked, exhibiting no further handedness change on CPL irradiation (d). Figure 6: Manipulation of supramolecular chirality entirely by light. The whole process of induction, control and locking of supramolecular chirality by CPL and CPUL from an achiral compound 1 containing TPA (yellow) and DA (red: non-polymerized, blue: polymerized) moieties is schematically depicted. Irradiation with CPL induces self-assembly of 1 with control over handedness ( a ) and the handedness can be reversibly switched by irradiating with the counter CPL ( b ). Photopolymerization of the DA moieties by CPUL irradiation knits the self-assembled structure to produce a covalently joined nano-object ( c ) and the supramolecular chirality is permanently locked, exhibiting no further handedness change on CPL irradiation ( d ). Full size image Conductivity measurement As it was previously demonstrated that one-dimensional self-assembled structures of TPA derivatives formed by photoirradiation have conductivity along the assembly axis [19] , [46] , [47] , [48] , we also investigated the current–voltage relationship of the self-assembled structures of 1 , to determine the effect of supramolecular chirality and photopolymerization of the DA moieties on conductivity ( Supplementary Fig. 12 ). When the DCE solution of 1 was placed on a gold nanogap of 500 nm with 2 V of continuous potential difference and visible light was turned on, current between the nanogap increased by approximately four orders of magnitude after 100 s giving conductivity of 1.4 S cm −1 , which was comparable to other conducting organic materials. Consistent with the previous result, conductivity was maintained in the solution state under light exposure (that is, as long as radicals were being continuously generated) and could even be reversibly controlled by turning the light on and off ( Supplementary Fig. 12b ). Interestingly, the conductivity of the photopolymerized aggregates was similar to the non-polymerized ones, and was also modulated by light irradiation, despite the fact that the covalently joined self-assembled structure could not dissociate under any circumstances ( Supplementary Fig. 12c ). The result suggests photopolymerization of the DA moieties does not affect the electrical properties of the TPA moieties and the key to conductivity is maintaining stable radicals at the nitrogen atom. We developed a light-controlled self-assembling system that can evolve and arrest supramolecular chirality following the information encoded in CPL. Our results suggest that the chiral bias generated by CPL can not only be transferred to a supramolecular level but also considerably amplified when combined with a self-assembly process, which preferentially incorporates one enantiomer into the self-assembled helical structure with specific handedness dictated by the rotational direction of CPL. This methodology provides complete control over the entire evolutionary process of supramolecular chirality using light and will be useful for future applications such as chiral sensors and chiral discrimination. Materials 1-Hydroxybenzotriazole monohydrate (HOBT) (97%) and 1-(3-dimethylaminopropyl)-3-ethylcarbodiimide hydrochloride (EDC) (98%) were purchased from Tokyo Chemical Industry Co. Triethylamine (Et 3 N) (99.5%) was purchased from Sigma-Aldrich. N , N -Dimethylformamide (DMF) (99.5%) and DCE were purchased from Junsei Chemical Co., Ltd. All chemicals were used as received. Tris(4-aminophenyl)amine ( 2 ) [49] and trideca-4,6-diynoic acid ( 3 ) [50] were synthesized according to the literature procedures. Characterization 1 H and 13 C NMR spectroscopies were conducted using a Bruker Science Avance 400 MHz NMR spectrometer with the residual solvent signal as an internal reference. High-resolution mass spectroscopy was performed on a Bruker Daltonik microTOF-Q II mass spectrometer using electrospray ionization method. Elemental analysis was conducted using a Thermo Scientific FLASH 2000 series elemental analyser. FE-SEM was performed on a FEI company Nova 230 SEM. Samples were prepared on a silicon wafer by dropping DCE solution of 1 (2 mg ml −1 ) and evaporation of the solvent. The samples were coated with Au before imaging. Transmission electron microscopy was performed on a JEOL Ltd. JEM-2100F 200 kV field-emission transmission electron microscope. Samples were prepared on a 300-mesh carbon film by dropping DCE solution of 1 (2 mg ml −1 ) and evaporation of the solvent. The samples were stained by exposing ruthenium tetroxide vapour before imaging. XRD patterns were obtained with a Rigaku D/MAX-2500 X-ray diffractometer with scan speed of 2° per minute and sampling width of 0.01°. Cu K α ( λ =0.154 nm) was used as a light source. Samples for wide-angle XRD were prepared by spin coating of DCE solution of 1 (2 mg ml −1 ) on a glass substrate. For small-angle XRD experiments, solid obtained by evaporation of the DCE solution was ground and loaded on a sample holder using carbon tape. Fourier-transform Raman spectra were obtained on an ARAMIS Horiba Jobin Yvon spectrometer with 633 nm He-Ne laser source. Samples were prepared by spin coating of DCE solution of 1 . Dynamic light scattering measurement was performed on a Brookhaven Instruments Corp. 90Plus/BI-MAS particle size analyser at wavelength of 658 nm with scattering angle of 90 °. Samples were prepared by dilution of DCE solution of 1 (2 mg ml −1 ) into 1/20 concentration (0.1 mg ml −1 ). CD spectra were obtained using Jasco Inc., Jasco-815 Spectropolarimeter equipped with temperature controller. Measurement was conducted with DCE solution of 1 in a 0.2-nm quarts cell at −10 °C using scan speed of 200 nm min −1 and sampling width of 1 nm. FT infrared spectroscopy was performed by attenuated total reflection infrared spectroscopy with a Bruker Science Platinum-ATR Alpha FT-infrared spectrometer. Samples were prepared by dropping the DCE solution of 1 (2 mg ml −1 ) on a sample window. Synthesis of tris(4-trideca-4,6-diynamidophenyl)amine ( 1 ) Tris(4-aminophenyl)amine (0.209 g, 0.720 mmol), trideca-4,6-diynoic acid (0.520 g, 2.520 mmol) and 1-hydroxybenzotriazole monohydrate (0.486 g, 3.60 mmol) were dissolved in 50 ml of N , N -dimethylformamide. The reaction mixture was stirred at 0 °C for 30 min. Next, 1-(3-dimethylaminopropyl)-3-ethylcarbodiimide hydrochloride (0.690 g, 3.60 mmol) and triethylamine (0.364 g, 3.60 mmol) were added into the solution and the reaction mixture was warmed up to room temperature (RT). After stirring for 12 h, the reaction mixture was poured into brine and extracted with tetrahydrofuran. The organic layer was washed with water, dried over anhydrous MgSO 4 and condensed in a rotary evaporator, to yield a crude product. Column chromatography on silica gel with tetrahydrofuran/hexane 1:1 as an eluent and recrystallization in ethanol produced pure 1 as a red solid (0.219 g, yield 35.57%). Electrospray ionization–mass spectrometry, m/e 877.50 for [M+Na] + (Calcd: 854.51). δ H (400 MHz, DMSO- d 6 ; p.p.m.) 9.89 (3H, s , N H CO), 7.44 (6H, d , J =8.9 Hz, Ar), 6.87 (6H, d , J =8.8 Hz, Ar), 2.54 (12H, t , J =7.2 Hz, C≡CC H 2 ), 2.23 (6H, t , J =6.9 Hz, COC H 2 ), 1.40 (6H, p , J =6.7 Hz, C≡CCH 2 C H 2 ), 1.29 (6H, m , C H 2 CH 3 ), 1.20 (12H, m , CH 2 C H 2 C H 2 CH 2 ), 0.80 (9H, t , J =6.6 Hz, C H 3 ). δ C (100 MHz, DMSO- d 6 ; p.p.m.) 168.66, 142.78, 133.95, 123.61, 120.35, 78.38, 76.99, 65.43, 65.24, 34.66, 30.63, 27.85, 27.63, 21.95, 18.26, 14.80, 13.88. Anal. Calcd for C 57 H 66 N 4 O 3 : C 80.06, H 7.78, N 6.55; Found: C 80.08, H 7.82, N 6.65. Photoinduced self-assembly of 1 DCE solution of 1 (2 mg ml −1 ) was irradiated with a hand-held lamp having 400–600 nm range of wavelength and 450 nm of maximum intensity with power of 1.5 W at RT. CPL was produced by placing a linear polarizer and quarter-lambda wave plate in front of the light source. The lamp was placed at 3 cm from each sample in every experiment and external light was prevented to leak into experimental samples. DFT calculation DFT calculation was conducted using Gaussian 09 (ref. 51 ). The long-range corrected hybrid density functional with damped atom–atom dispersion correction, ω B97X-D, was used [52] . This functional can handle π - π interaction empirically and have been successfully used to model polymer structures with large number of atoms [53] , [54] , [55] . The 6-31G* basis set was used to describe atomic orbitals. For efficient calculation, we simplified the molecular structure by assuming a planar C3 symmetric structure for the TPA moiety and substituting the side chains with n -pentyl groups and then optimized its pentamer structure. A unit positive charge was added to the pentamer and the doublet spin state was calculated to account for the electronic effect of the cationic radical species in the aggregate. The optimized pentamer structure is shown in Supplementary Fig. 5 . The trimer structure shown in Fig. 2 was obtained from the optimized pentamer by removing the terminal molecule, to avoid unrealistic end group contribution and illustrate a proper arrangement in the middle of the stack. In the trimer, the degree of rotation per molecule was 12.1° on average and intermolecular distance between the TPA moieties was estimated to be 0.436 nm, which was comparable to the spacing of 0.42 nm obtained by the XRD analysis. We also note that amide hydrogen bonding between the alkyl chains of the adjacent molecules reinforces the assembly. The intermolecular distance between the terminal methyl carbons was calculated to be an average 0.454 nm, suggesting the feasibility of topochemical polymerization of the adjacent DA groups by light [56] , [57] , [58] . CD spectra were simulated based on the time-dependent DFT method [59] . The trimer geometry was employed to calculate the excitation energy assuming that the geometric change during the electronic excitation would be negligible. The same functional ω B97X-D was used to calculate the electronic excitation energy, but the size of the basis set was reduced to 3-21G* due to the computational cost. Only singlet excited states was considered and the number of roots for the singlet state was 30. The raw Gaussian 09 output file was processed using GaussSum [60] , to yield CD spectra. Conductivity measurement Au nanogap was fabricated as follows. On the thermally grown SiO 2 /Si wafer cleaned by a mixture of H 2 SO 4 and H 2 O 2 for 10 min, Cr/Au was thermally evaporated at 1 × 10 −6 torr to form a Cr layer with 10 nm thick and a Au layer with 40 nm thick, respectively. By conventional photolithography, metal lines with width of 44 μm were patterned. After then, a focused ion beam (FB-2100, Hitachi, Co.) was used to form a 500-nm gap. In light and electromagnetic wave shielded probe station at RT, the fabricated nanogap covered with DCE solution of 1 was placed in a sealed vessel made of quartz. Visible light (1.5 W) were exposed to samples through the quartz vessel and 2 V of continuous potential difference was held across the nanogap. Photopolymerization of assembled structure of 1 between nanogap was conducted by irradiation of ultraviolet from 8 W hand-held ultraviolet lamp at the distance of 3 cm through the quartz vessel. The current–voltage ( I – V ) relationships were obtained by precision semiconductor parameter analyser (HP 4156A, Hewlett Packard Co.). How to cite this article: Kim, J. et al . Induction and control of supramolecular chirality by light in self-assembled helical nanostructures. Nat. Commun. 6:6959 doi: 10.1038/ncomms7959 (2015).